BRCA1 and CtIP suppress long-tract gene conversion between sister chromatids BRCA1 controls early steps of the synthesis-dependent strand annealing (SDSA) pathway of homologous recombination, but has no known role following Rad51-mediated synapsis. Here we show that BRCA1 influences post-synaptic homologous recombination events, controlling the balance between short- (STGC) and long-tract gene conversion (LTGC) between sister chromatids. Brca1 mutant cells reveal a bias towards LTGC that is corrected by expression of wild-type but not cancer-predisposing BRCA1 alleles. The LTGC bias is enhanced by depletion of CtIP but reversed by inhibition of 53BP1, implicating DNA end resection as a contributor to the STGC/LTGC balance. The impact of BRCA1/CtIP loss on the STGC/LTGC balance is abolished when the second (non-invading) end of the break is unable to support termination of STGC by homologous pairing (annealing). This suggests that BRCA1/CtIP-mediated processing of the second end of the break controls the annealing step that normally terminates SDSA, thereby suppressing the error-prone LTGC outcome. Double-strand breaks (DSBs) are dangerous DNA lesions, the misrepair of which can promote genomic instability and cancer [1] , [2] . Chromosome breakage in proliferating cells commonly arises in the S phase of the cell cycle during replication across a damaged DNA template [3] , [4] , [5] . Such DSBs can be repaired by sister chromatid recombination (SCR), a potentially error-free pathway in which the broken chromosome uses the neighbouring sister chromatid as a template for repair by homologous recombination (HR). The major hereditary breast/ovarian cancer predisposition genes, BRCA1 and BRCA2 , have established functions in HR. A long-standing hypothesis proposes that BRCA1 and BRCA2 execute tumour suppressor functions in SCR [6] . HR entails resection of the DNA end to single-stranded (ss) DNA, on which Rad51 polymerizes to form a Rad51-ssDNA nucleoprotein filament [7] , [8] , [9] . This filament conducts a homology search by invading neighbouring DNA duplexes and base-pairing with a homologous donor such as the neighbouring sister chromatid. A DNA polymerase extends the invading 3′ DNA end (the ‘nascent’ strand). In somatic eukaryotic cells, the major HR pathway is ‘synthesis-dependent strand annealing’ (SDSA), a non-crossover pathway in which termination occurs by annealing of the displaced nascent strand with complementary sequences in the resected second end of the broken chromosome [7] . Gene conversion can occur if the homologous donor differs in sequence from the broken chromosome. Studies in yeast indicate the existence of at least two distinct copying mechanisms in HR, which differ in their fidelity. In Saccharomyces cerevisiae , the majority of somatic gene conversions entail SDSA-mediated copying of a short (<200 bp) stretch of information from the donor. An alternative pathway termed break-induced replication (BIR) can mediate long gene conversions in yeast, potentially extending the nascent strand as far as the end of the chromosome [10] , [11] , [12] , [13] . BIR may entail formation of a bona fide replication fork at the site of recombination and requires both leading and lagging strand synthesis. In yeast, BIR can arise in response to one-ended invasions occurring without a homologous second end, a key trigger being the failure of the second end of the DSB to effect termination of HR [14] , [15] , [16] , [17] . To what extent BIR operates in mammalian cells is not well understood. In mammalian cells, gene conversions typically extend less than 100 bp (‘short-tract’ gene conversion—STGC) [18] , [19] , [20] . A small proportion of HR events entail ‘long-tract’ gene conversion (LTGC), in which nascent strand synthesis extends several kilobases prior to termination [21] , [22] , [23] . LTGC is an error-prone HR outcome, causing tandem gene duplication and, rarely, multi-copy gene amplification [22] . Mammalian cells lacking any one of the Rad51 paralogues XRCC3, Rad51C or XRCC2 reveal a specific defect in STGC and marked bias in favour of LTGC, which accounts for ~25% of all gene conversions in Rad51 paralogue-deficient cells [23] , [24] , [25] . Increased proportions of LTGC-type products were also observed in a Brca2 mutant hamster cell line and in Nbs1 null chicken DT40 lymphoblastoid cells [26] , [27] . The identity of other genes that regulate the balance between STGC and LTGC is unknown. BRCA1 supports DNA end resection via its interactions with CtIP (C-terminus-binding protein of adenovirus E1A-interacting protein) and the Mre11/Rad50/NBS1 (MRN) complex to generate ssDNA that serves as substrate for BRCA2-mediated Rad51 nucleoprotein filament formation [28] . BRCA1 also interacts with BRCA2 via the bridging protein, PALB2 (partner and localizer of BRCA2), as well as with BACH1/BRIP1 and the chromatin-associated RAP80 complex [29] , [30] , [31] , [32] . Deletion of 53bp1 , a gene implicated in NHEJ and in the suppression of DNA end resection, rescues the Brca1 mutant phenotype in the mouse, suggesting a primary role for BRCA1 in DNA end resection [33] . Thus, the known functions of BRCA1 in HR are restricted to the early steps preceding Rad51-mediated synapsis. To test whether BRCA1 influences later HR steps, we studied its contribution to STGC and LTGC between sister chromatids, induced by a site-specific chromosomal DSB. We show here that loss of BRCA1 or CtIP skews HR in favour of the LTGC outcome; this is reversed by wild-type BRCA1 but not by certain cancer-predisposing BRCA1 alleles. The influence of BRCA1 and CtIP on the STGC/LTGC balance is lost when the second (non-invading) end of the DSB is unable to support termination of STGC by annealing. We conclude that BRCA1/CtIP controls the balance between STGC and LTGC by acting on the second end of the DSB to support the annealing step that normally terminates STGC. These findings suggest that a defect in the early stages of HR, caused by loss of BRCA1 function, can translate into a defect in HR termination, skewing this process towards error-prone repair at the expense of error-free repair. A reporter for rapid flow cytometric analysis of LTGC We previously described a SCR reporter to simultaneously measure STGC and LTGC between sister chromatids [22] , [34] . Expression of the rare-cutting homing endonuclease I-SceI [35] induces a site-specific DSB within a mutant copy of the gene encoding enhanced green fluorescent protein (E-GFP, here termed ‘GFP’). Recombination between the broken GFP copy and neighboring 5′ truncated GFP sequences produces wild-type GFP by gene conversion, and the cell changes from GFP – to GFP + . In the original reporter, duplication of a cassette during LTGC enabled positive selection of LTGC through expression of a wild-type antibiotic resistance gene [22] . We re-fashioned this reporter so that the cassette duplicated during LTGC encodes the monomeric red fluorescent protein RFP1.3 (here termed ‘RFP’; Fig. 1a ) [36] . Briefly, we divided the RFP cDNA into two artificial exons (‘A’ and ‘B’ in Fig. 1a ), with appropriate splice donor and acceptor sequences. The RFP exons were placed ‘head to toe’ between the two GFP copies of the reporter so that transcription of exon A within the unmodified (parental) reporter will not lead to expression of wild-type RFP . During STGC, the cell becomes GFP + RFP – ( Fig. 1a , outcome no. 1). In contrast, LTGC typically generates three GFP copies ( GFP triplication) by SCR and duplicates the RFP cassette ( Fig. 1a , outcome no. 2). Splicing between exon A of the first cassette and exon B of the second generates wt RFP mRNA and the cell becomes GFP + RFP + . A minority of LTGCs duplicate RFP exon B but terminate prior to triplication of the GFP copies (‘early termination’ of LTGC—nascent strand extension of between 1,252 bp and 3.4 kb). 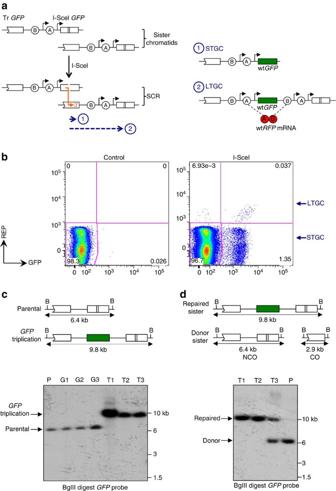Figure 1: RFP-SCR reporter for quantifying short-tract and long-tract gene conversion. (a) Structure of the RFP-SCR reporter. Circles A and B: 5′ and 3′ artificialRFPexons. Black arrows: promoters. TrGFP: 5′ truncatedGFP. Orange arrow: Rad51-mediated strand invasion (3′ end marked with arrow head). Blue dashed arrow 1: short-tract gene conversion (STGC); 2: long-tract gene conversion (LTGC). LTGC generates wtRFPmRNA. (b) I-SceI -induced HR products inBrca1fl/mutRFP-SCR reporter ES cells. Note GFP+RFP–(STGC) and GFP+RFP+(LTGC) populations. (c) Southern blot analysis of HR products. ‘Parental’: unrearranged RFP-SCR reporter; ‘GFPtriplication’: LTGC or crossover product. B: BglII sites. Boxes areGFPcopies; green box is wtGFP.RFPcassette is not shown. Gel lanes—P: parental; G1–G3: GFP+RFP–STGC products; T1–T3: GFP+RFP+‘GFPtriplication’ products. (d) Donor sister chromatid structure distinguishes non-crossover (NCO) from crossover (CO) ‘GFPtriplication’ outcome. Cartoon elements as in (c). Gel lanes—T1–T3: GFP+RFP+clones (different from panelc); P: parental. Note the unrearranged donor sister in T3, implying a NCO mechanism (LTGC). Figure 1: RFP-SCR reporter for quantifying short-tract and long-tract gene conversion. ( a ) Structure of the RFP-SCR reporter. Circles A and B: 5′ and 3′ artificial RFP exons. Black arrows: promoters. Tr GFP : 5′ truncated GFP . Orange arrow: Rad51-mediated strand invasion (3′ end marked with arrow head). Blue dashed arrow 1: short-tract gene conversion (STGC); 2: long-tract gene conversion (LTGC). LTGC generates wt RFP mRNA. ( b ) I-SceI -induced HR products in Brca1 fl/mut RFP-SCR reporter ES cells. Note GFP + RFP – (STGC) and GFP + RFP + (LTGC) populations. ( c ) Southern blot analysis of HR products. ‘Parental’: unrearranged RFP-SCR reporter; ‘ GFP triplication’: LTGC or crossover product. B: BglII sites. Boxes are GFP copies; green box is wt GFP . RFP cassette is not shown. Gel lanes—P: parental; G1–G3: GFP + RFP – STGC products; T1–T3: GFP + RFP + ‘ GFP triplication’ products. ( d ) Donor sister chromatid structure distinguishes non-crossover (NCO) from crossover (CO) ‘ GFP triplication’ outcome. Cartoon elements as in ( c ). Gel lanes—T1–T3: GFP + RFP + clones (different from panel c ); P: parental. Note the unrearranged donor sister in T3, implying a NCO mechanism (LTGC). Full size image We targeted a single copy of the RFP-SCR reporter to the ROSA26 locus of the mouse embryonic stem (ES) cell line 11CO/47T [37] , in which one Brca1 allele is truncated and the second can be conditionally inactivated by Cre-mediated recombination (here termed ‘ Brca1 fl/mut ’ cells, described in detail below; see Methods). Transfection of Brca1 fl/mut RFP-SCR reporter cells with I-SceI elicited GFP + RFP – and GFP + RFP + products ( Fig. 1b ). We used fluorescence-activated cell sorting (FACS) to sort single GFP + RFP – or GFP + RFP + cells from I-SceI-transfected samples, prepared genomic DNA (gDNA) from amplified clones and analysed the structure of the RFP-SCR reporter by Southern blotting. All FACS-sorted GFP + RFP – clones revealed a structurally unrearranged RFP-SCR reporter, consistent with STGC (examples in Fig. 1c , lanes G1–G3). In contrast, >95% of GFP + RFP + clones revealed rearrangements of the RFP-SCR reporter characteristic of LTGC (examples in Fig. 1c , lanes T1–T3; more detailed mapping in Supplementary Fig. S1 ). Donor sister chromatid distinguishes LTGC from crossing over The ‘ GFP triplication’ outcome could arise by either LTGC or crossing over. In LTGC, the donor sister chromatid is unaltered, whereas crossing over results in loss of one GFP copy from the donor sister ( Fig. 1d ). Previous work established that crossing over is suppressed in somatic cells [21] , [23] . To distinguish these mechanisms, we adapted a strategy we used previously to capture the donor sister chromatid in the context of I-SceI-induced HR [23] . We found that a small fraction of sorted I-SceI-induced GFP + RFP + cells were mixed colonies, in which the GFP + RFP + cell had been sorted subsequent to an LTGC event but prior to the ensuing mitosis. Such clones should therefore contain HR products from both sister chromatids. We identified four such mixed colonies; all (4/4) revealed the ‘ GFP triplication’ outcome and an unrearranged donor (for example, lane T3 in Fig. 1d ). Although the number of events detected was small, the consistently unrearranged donor suggests that LTGC is the major mechanism underlying the ‘ GFP triplication’ outcome. 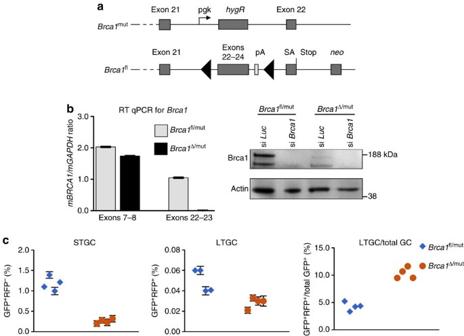Figure 2: Bias in favour of LTGC inBrca1Δ/mutES cells. (a)Brca1gene structure inBrca1fl/mutES cells.Brca1mutallele encodes the truncated product.Brca1flallele converts to ‘Brca1Δ’ following Cre-mediated recombination. Grey boxes:Brca1exons; black triangles:loxPsites; SA: splice acceptor. (b) Analysis ofBrca1gene products inBrca1fl/mutandBrca1Δ/mutES cells. Left panel: RT qPCR analysis of mRNA exon boundaries. Note the loss of exon 22–23 signal inBrca1Δ/mutcells. Right panel: Brca1 protein levels inBrca1fl/mutandBrca1Δ/mutES cells following transfection with siRNA against luciferase (siLuc) or Brca1 (siBrca1). Note the persistent Brca1 product inBrca1Δ/mutES cells, consistent with hypomorphic status. (c) I-SceI -induced HR in four independentBrca1fl/mut(blue diamonds) and four independentBrca1Δ/mut(orange circles) Cre-treated RFP-SCR reporter ES cell clones. Each point shows the mean of quadruplicate samples for one independent clone. Error bars: standard error of the mean (s.e.m.) in this and all subsequent figures. STGC, LTGC and LTGC/Total GC products are shown. In the last panel, error bars are smaller than the symbols. Bias in favour of LTGC in Brca1 Δ/mut RFP-SCR reporter cells Figure 2a depicts the structure of the two Brca1 alleles in Brca1 fl/mut ES cell line 11CO/47T [37] . One allele ( Brca1 mut ) encodes a C-terminally truncated Brca1 gene product (lacking a functional BRCT repeat). The second allele ( Brca1 fl ) contains mouse Brca1 cDNA sequences corresponding to exons 22–24 flanked by loxP sites ( Fig. 2a ). Cre-mediated deletion converts the functionally wt Brca1 fl allele to a mutant allele ( Brca1 Δ ) that encodes a C-terminally truncated Brca1 product similar to that encoded by the Brca1 mut allele. We transduced Brca1 fl/mut RFP-SCR reporter ES cells with Cre-encoding adenovirus and screened clones for Brca1 inactivation by real-time qPCR ( Fig. 2b and Methods). We identified Brca1 -deleted clones and others that remained undeleted. Brca1 null ES cells are unviable [38] ; very likely, Brca1 mut and Brca1 Δ are hypomorphic alleles. Consistent with this, we detected by immunoblotting Brca1 gene products at low abundance in Brca1 Δ/mut ES cell clones. These Brca1 proteins were further depleted by siRNA directed to Brca1 ( Fig. 2b ). Figure 2: Bias in favour of LTGC in Brca1 Δ/mut ES cells. ( a ) Brca1 gene structure in Brca1 fl/mut ES cells. Brca1 mut allele encodes the truncated product. Brca1 fl allele converts to ‘ Brca1 Δ ’ following Cre-mediated recombination. Grey boxes: Brca1 exons; black triangles: loxP sites; SA: splice acceptor. ( b ) Analysis of Brca1 gene products in Brca1 fl/mut and Brca1 Δ/mut ES cells. Left panel: RT qPCR analysis of mRNA exon boundaries. Note the loss of exon 22–23 signal in Brca1 Δ/mut cells. Right panel: Brca1 protein levels in Brca1 fl/mut and Brca1 Δ/mut ES cells following transfection with siRNA against luciferase (si Luc ) or Brca1 (si Brca1 ). Note the persistent Brca1 product in Brca1 Δ/mut ES cells, consistent with hypomorphic status. ( c ) I-SceI -induced HR in four independent Brca1 fl/mut (blue diamonds) and four independent Brca1 Δ/mut (orange circles) Cre-treated RFP-SCR reporter ES cell clones. Each point shows the mean of quadruplicate samples for one independent clone. Error bars: standard error of the mean (s.e.m.) in this and all subsequent figures. STGC, LTGC and LTGC/Total GC products are shown. In the last panel, error bars are smaller than the symbols. Full size image To determine whether loss of wt Brca1 influences the balance between STGC and LTGC, we transfected, in parallel, the above-noted Cre-treated Brca1 fl/mut and Brca1 Δ/mut RFP-SCR reporter clones with either I-SceI plasmid or empty vector and quantified HR products ( Fig. 2c ; see Methods). In all experiments described here, clones that were treated with empty vector control revealed typical background levels of ~0.03% GFP + RFP – and of <0.001% GFP + RFP + , with at least 200,000 events counted per sample. All I-SceI-induced HR measurements were corrected for background events and for I-SceI transfection efficiency (see Methods), the latter being typically between 65 and 85%; neither measurement varied with Brca1 status. We compared four independent Cre-treated Brca1 Δ/mut and Brca 1 fl/mut RFP-SCR reporter clones. All four Brca1 Δ/mut clones revealed reduced frequencies of HR, as expected [39] , but only a modest reduction in LTGC ( Fig. 2c ). The ratio GFP + RFP + /Total GFP + estimates the probability that an I-SceI-induced GFP + HR event will resolve as LTGC. This probability was elevated ~2-fold in Brca1 Δ/mut cells in comparison with isogenic Brca1 fl/mut cells ( Fig. 2c , lower panel). Thus, loss of wt Brca1 skews HR in favour of LTGC. We studied the structure of the reporter in I-SceI-induced GFP + RFP + clones derived from Brca1 Δ/mut cells and isogenic Cre-treated Brca1 fl/mut cells by Southern blotting. As noted above, most LTGCs entail ‘ GFP triplication’ ( Fig. 1a , outcome no. 2), while a minority terminate within the reporter subsequent to duplication of RFP exon B (‘early termination’) [21] , [22] , [23] , [34] . In Brca1 fl/mut cells, 58/65 (89.2%) GFP + RFP + clones entailed GFP triplication while 4/65 (6.1%) GFP + RFP + clones revealed early termination of LTGC. In Brca1 Δ/mut cells, 28/29 (96.6%) of GFP + RFP + clones were GFP triplications and 1/29 (3.4%) revealed early termination of LTGC. Thus, loss of Brca1 does not grossly alter the types of LTGC detected. Capture and analysis of the donor sister chromatid in mixed I-SceI-induced GFP + RFP + clones sorted from Brca1 Δ/mut cells revealed an intact donor sister chromatid in 3/3 GFP triplication clones examined, confirming that they arose by a non-crossover mechanism, that is, by LTGC. Wild-type BRCA1 rescues the HR defects of Brca1 Δ/mut cells The bias in favour of LTGC noted in Brca1 Δ/mut cells could reflect secondary/compensatory responses to Brca1 loss. To test this, we transiently co-transfected Brca1 Δ/mut and, in parallel, Brca1 fl/mut RFP-SCR reporter clones with wt human BRCA1 and I-SceI and measured HR. Human BRCA1 can restore normal development to Brca1 null mice [40] . Notably, wild-type BRCA1 complemented the STGC defect and corrected the LTGC bias in Brca1 Δ/mut cells, but had little impact on any HR measurements in Brca1 fl/mut cells ( Fig. 3 ). In contrast to wt BRCA1 , expression of cancer-predisposing BRCA1 alleles encoding point mutant products affecting the RING domain (C61G, C64G; Fig. 3a–c ) or the tandem BRCT repeat (P1749R, M1775R; Fig. 3d–f ) had no impact on HR in Brca1 Δ/mut cells, despite levels of BRCA1 mutant gene expression higher than those of wt BRCA1 ( Supplementary Fig. S2 ; at the low levels of exogenous BRCA1 used in these experiments, we were unable to detect the hBRCA1 protein). These results suggest that a tumour suppressor function of BRCA1 specifically enforces STGC in favour of LTGC. 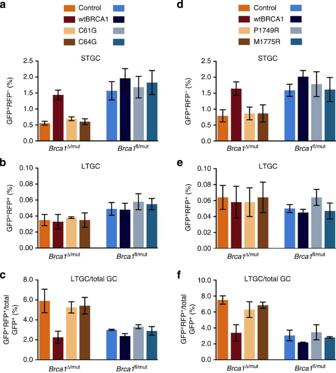Figure 3: Wild type but not cancer-predisposing mutant alleles of humanBRCA1complement the STGC defect inBrca1Δ/mutES cells. Data pooled from three independent experiments, each performed with triplicate samples. Error bars: s.e.m.,n=3. (a) I-SceI -induced STGC inBrca1Δ/mutandBrca1fl/mutRFP-SCR reporter ES cells transiently transfected with I-SceI and with control (orange or blue), wtBRCA1(maroon or dark blue),BRCA1C61G (apricot or grey) orBRCA1C64G (brown or teal).Brca1Δ/mutcells: wtBRCA1versus control: pairedt-test:P=0.01. OtherBRCA1alleles versus control: not significant (NS).Brca1fl/mutcells: all test samples versus control: NS. (b) I-SceI -induced LTGC in the experiment shown in (a). All test samples versus control: NS. (c) Ratio of I-SceI -induced LTGC/overall GC in the experiment shown in (a) and (b).Brca1Δ/mutcells: wtBRCA1versus control: pairedt-test:P=0.04. OtherBRCA1alleles versus control: NS.Brca1fl/mutcells: all test samples versus control: NS. (d) Similar to (a), but withBRCA1P1749R (apricot or grey) orBRCA1M1775R (brown or teal).Brca1Δ/mutcells: wtBRCA1versus control: pairedt-test:P=0.05. OtherBRCA1alleles versus control: NS.Brca1fl/mutcells: all test samples versus control: NS. (e) I-SceI-induced LTGC events in the experiment shown in (d). All test samples versus control: NS. (f) Ratio of I-SceI-induced LTGC/overall GC in the experiment shown in (d) and (e).Brca1Δ/mutcells: wtBRCA1versus control: pairedt-test:P=0.03. OtherBRCA1alleles versus control: NS.Brca1fl/mutcells: all test samples versus control: NS. Figure 3: Wild type but not cancer-predisposing mutant alleles of human BRCA1 complement the STGC defect in Brca1 Δ/mut ES cells. Data pooled from three independent experiments, each performed with triplicate samples. Error bars: s.e.m., n =3. ( a ) I-SceI -induced STGC in Brca1 Δ/mut and Brca1 fl/mut RFP-SCR reporter ES cells transiently transfected with I-SceI and with control (orange or blue), wt BRCA1 (maroon or dark blue), BRCA1 C61G (apricot or grey) or BRCA1 C64G (brown or teal). Brca1 Δ/mut cells: wt BRCA1 versus control: paired t -test: P =0.01. Other BRCA1 alleles versus control: not significant (NS). Brca1 fl/mut cells: all test samples versus control: NS. ( b ) I-SceI -induced LTGC in the experiment shown in ( a ). All test samples versus control: NS. ( c ) Ratio of I-SceI -induced LTGC/overall GC in the experiment shown in ( a ) and ( b ). Brca1 Δ/mut cells: wt BRCA1 versus control: paired t -test: P =0.04. Other BRCA1 alleles versus control: NS. Brca1 fl/mut cells: all test samples versus control: NS. ( d ) Similar to ( a ), but with BRCA1 P1749R (apricot or grey) or BRCA1 M1775R (brown or teal). Brca1 Δ/mut cells: wt BRCA1 versus control: paired t -test: P =0.05. Other BRCA1 alleles versus control: NS. Brca1 fl/mut cells: all test samples versus control: NS. ( e ) I-SceI-induced LTGC events in the experiment shown in ( d ). All test samples versus control: NS. ( f ) Ratio of I-SceI-induced LTGC/overall GC in the experiment shown in ( d ) and ( e ). Brca1 Δ/mut cells: wt BRCA1 versus control: paired t -test: P =0.03. Other BRCA1 alleles versus control: NS. Brca1 fl/mut cells: all test samples versus control: NS. Full size image The above experiments implicate both the BRCA1 N-terminal RING and C-terminal BRCT domains in STGC and in preventing an LTGC bias during HR. The BRCA1 RING domain mediates constitutive heterodimerization with BARD1 in vertebrate cells and BRCA1 RING domain mutations C61G and C64G disrupt the BRCA1−BARD1 interaction, while retaining some residual function [41] , [42] . We used transient transfection of siRNA to deplete either Brca1 or Bard1 in Brca1 Δ/mut or Brca1 fl/mut RFP-SCR reporter cells in conjunction with I-SceI transfection (see Methods). Consistent with the hypomorphic status of Brca1 Δ/mut cells, siRNA-mediated depletion of Brca1 reduced HR in both Brca1 Δ/mut and Brca1 fl/mut cells ( Supplementary Fig. S3 ). siRNA-mediated depletion of Brca1 also further exacerbated the LTGC bias in Brca1 Δ/mut cells, but produced only minimal alterations in the STGC/LTGC balance in Brca1 fl/mut cells. A similar pattern was observed following siRNA-mediated depletion of Bard1 ( Supplementary Fig. S3 ). The limited impact of Brca1 -specific siRNA on the STGC/LTGC balance in Brca1 fl/mut cells may reflect the residual activity of wt Brca1 in siRNA-depleted Brca1 fl/mut cells, and indicates that siRNA-mediated methods for perturbing the LTGC/STGC balance have false-negative rates, as was noted previously [23] . CtIP regulates the balance between STGC and LTGC At least three major distinct DNA damage response complexes interact with the BRCA1/BARD1 heterodimer via the BRCA1 tandem BRCT repeat, which they bind in a mutually exclusive fashion. These are (direct BRCA1 interactors underlined): CCDC98/Abraxas , RAP80, BRCC36, BRCC45, and MERIT40; BACH1 and TopBP1; and CtIP [29] , [30] , [31] . These interactions are disabled by BRCA1 BRCT mutations P1749R and M1775R. The failure of these BRCA1 BRCT mutants to restore a normal STGC/LTGC balance to Brca1 Δ/mut cells therefore suggested possible roles for CtIP, BACH1 or Abraxas/Rap80 as regulators of the STGC/LTGC balance. Bach1 depletion reduced HR in both Brca1 Δ/mut and Brca1 fl/mut cells [43] ( Supplementary Fig. S4 ). This suggests that at least part of Bach1’s HR function is independent of its interaction with Brca1. Rap80 depletion caused an unexpected reduction in HR in both Brca1 Δ/mut and Brca1 fl/mut cells, in contrast to recent findings of several groups in cells with normal BRCA1 function [32] , [44] , [45] . We do not understand the reason for this difference; however, Rap80 depletion was found to reduce HR in one other study, suggesting that Rap80’s function in HR is context-dependent [46] . siRNA-mediated depletion of CtIP, using either a single siRNA or SMARTpool siRNAs of non-overlapping specificity with the single CtIP siRNA, reduced HR in both Brca1 Δ/mut and Brca1 fl/mut cells—indicating that CtIP, like Bach1, can function in HR independent of its Brca1 interaction. siRNA-mediated depletion of BACH1 or Rap80 revealed exactly proportional alterations in I-SceI-induced STGC and LTGC in both Brca1 Δ/mut and Brca1 fl/mut cells ( Supplementary Fig. S4 ). In contrast, surprisingly, depletion of CtIP biased HR in favour of LTGC in both Brca1 Δ/mut and Brca1 fl/mut cells ( Fig. 4a–c ). 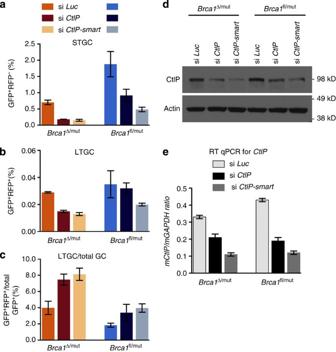Figure 4: CtIP controls the balance between LTGC and STGC. Data pooled from three independent experiments, each performed with triplicate samples. Error bars: s.e.m.,n=3. (a) I-SceI-induced STGC inBrca1Δ/mutandBrca1fl/mutRFP-SCR reporter ES cells co-transfected with I-SceI and with control Luciferase siRNA (siLuc, orange or blue), single CtIP siRNA (siCtIP, maroon or dark blue) or CtIP SMARTpool (siCtIP-smart, apricot or grey). Pairedt-test versus siLucinBrca1Δ/mutcells—siCtIP:P=0.03; siCtIP-smart:P=0.03; inBrca1fl/mutcells—siCtIP: NS. siCtIP-smart:P=0.05. (b) I-SceI-induced LTGC in the experiment shown in (a). Pairedt-test versus siLucinBrca1Δ/mutcells—siCtIP:P=0.002; siCtIP-smart:P=0.002; inBrca1fl/mutcells—siCtIP: NS. siCtIP-smart: NS. (c) Ratio of I-SceI-induced LTGC/overall GC in the experiment shown in (a) and (b). Pairedt-test versus siLucinBrca1Δ/mutcells—siCtIP:P=0.04; siCtIP-smart:P=0.04; inBrca1fl/mutcells—siCtIP: NS. siCtIP-smart:P=0.01. (d) Abundance of CtIP and actin (loading control) in the siRNA-treated cells used in (a), (b) and (c). (e) RT qPCR analysis ofCtIPmRNA in the siRNA-treated cells used in panels (a), (b) and (c). Figure 4: CtIP controls the balance between LTGC and STGC. Data pooled from three independent experiments, each performed with triplicate samples. Error bars: s.e.m., n =3. ( a ) I-SceI-induced STGC in Brca1 Δ/mut and Brca1 fl/mut RFP-SCR reporter ES cells co-transfected with I-SceI and with control Luciferase siRNA (si Luc , orange or blue), single CtIP siRNA (si CtIP , maroon or dark blue) or CtIP SMARTpool (si CtIP-smart , apricot or grey). Paired t -test versus si Luc in Brca1 Δ/mut cells — si CtIP : P =0.03; si CtIP-smart : P =0.03; in Brca1 fl/mut cells — si CtIP : NS. si CtIP-smart : P =0.05. ( b ) I-SceI-induced LTGC in the experiment shown in ( a ). Paired t -test versus si Luc in Brca1 Δ/mut cells — si CtIP : P =0.002; si CtIP-smart : P =0.002; in Brca1 fl/mut cells — si CtIP : NS. si CtIP-smart : NS. ( c ) Ratio of I-SceI-induced LTGC/overall GC in the experiment shown in ( a ) and ( b ). Paired t -test versus si Luc in Brca1 Δ/mut cells — si CtIP : P =0.04; si CtIP-smart : P =0.04; in Brca1 fl/mut cells — si CtIP : NS. si CtIP-smart : P =0.01. ( d ) Abundance of CtIP and actin (loading control) in the siRNA-treated cells used in ( a ), ( b ) and ( c ). ( e ) RT qPCR analysis of CtIP mRNA in the siRNA-treated cells used in panels ( a ), ( b ) and ( c ). Full size image CtIP regulates DNA end resection and is activated by the SIRT6 deacetylase [47] . Notably, Sirt6 depletion mimicked the effect of CtIP depletion, skewing HR in favour of LTGC, as did depletion of Exo1, an exonuclease implicated in DNA end resection ( Fig. 5 and Supplementary Fig. S5 ). Inhibition of 53BP1—an antagonist of Brca1 DNA end resection function [33] —using a previously characterized dominant-negative fragment of 53BP1 (ref. 48 ), specifically restored the STGC/LTGC balance to Brca1 Δ/mut cells but did not affect this balance in Brca1 fl/mut cells ( Fig. 5 ). This supports the idea that the LTGC bias in Brca1 Δ/mut cells is caused by a defect in DNA end resection. siRNA-mediated depletion of the early DSB response protein Mre11 had no impact on the STGC/LTGC balance, suggesting that not all resection proteins influence this balance ( Supplementary Fig. S5 ). We considered the possibility that the LTGC bias in ES cells depleted of CtIP might reflect altered cell cycle distribution [49] . However, cell cycle distribution did not vary between Brca1 Δ/mut or Brca1 fl/mut cells, whether they received siRNA directed to Luciferase, Bard1 or CtIP ( Supplementary Fig. S6 ). We determined whether the LTGC bias in cells lacking BRCA1/BARD1/CtIP is unique to mouse ES cells by studying human U2OS osteosarcoma cells carrying a single integrated copy of the RFP-SCR reporter (see Methods). Consistent with the above results, we observed a bias towards LTGC in U2OS cells depleted of BRCA1, BARD1 or CtIP ( Supplementary Fig. S7 ). Taken together, the results reveal a surprising and specific role for BRCA1/BARD1, CtIP and certain other DNA end resection complexes in controlling the balance between STGC and LTGC. 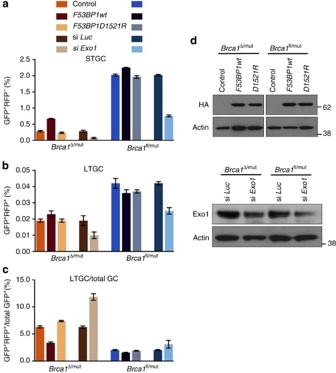Figure 5: Impact of overexpression of 53BP1 fragment and siRNA-mediated depletion of Exo1 on STGC and LTGC. Data pooled from three independent experiments, each performed with triplicate samples. Error bars: s.e.m.,n=3. (a) I-SceI-induced STGC frequencies inBrca1Δ/mutandBrca1fl/mutRFP-SCR reporter ES cells transiently co-transfected with I-SceI expression vector and with control vector (Control, orange or blue),F53BP1wtfragment (F53BP1wt, maroon or dark blue),F53BP1D1521Rfragment (D1521R, apricot or grey), Luciferase control siRNA (siLuc, brown or teal) or SMARTpool siRNA againstExo1(siExo1, light brown or sky blue). Pairedt-test versus control inBrca1Δ/mutcells—F53BP1wt:P=0.0001,D1521R: NS; inBrca1fl/mutcells—F53BP1wt: NS,D1521R: NS. Pairedt-test siLucversus siExo1inBrca1Δ/mutcells:P=0.00007, inBrca1fl/mutcells:P=0.0001. Error bars indicate s.e.m. throughout. (b) Frequency of I-SceI-induced LTGC events in the same experiment as in panel (a). Pairedt-test versus control inBrca1Δ/mutcells—F53BP1wt: NS,D1521R: NS; inBrca1fl/mutcells—F53BP1wt: NS,D1521R: NS. Pairedt-test siLucversus siExo1inBrca1Δ/mutcells:P=0.001, inBrca1fl/mutcells:P=0.007. (c) Ratio of I-SceI-induced GFP+RFP+/total GFP+frequencies (LTGC/overall GC, expressed as a percentage) from the same experiment as in panels (a) and (b). Pairedt-test against control inBrca1Δ/mutcells—F53BP1wt:P=0.0003,D1521R: NS; inBrca1fl/mutcells—F53BP1wt: NS,D1521R: NS. Pairedt-test siLucversus siExo1inBrca1Δ/mutcells:P=0.0001, inBrca1fl/mutcells:P=0.007. (d) Abundance of 53BP1 fragments, Exo1 and actin (loading control) in treatedBrca1Δ/mutandBrca1fl/mutRFP-SCR reporter ES cells in (a), (b) and (c). Figure 5: Impact of overexpression of 53BP1 fragment and siRNA-mediated depletion of Exo1 on STGC and LTGC. Data pooled from three independent experiments, each performed with triplicate samples. Error bars: s.e.m., n =3. ( a ) I-SceI-induced STGC frequencies in Brca1 Δ/mut and Brca1 fl/mut RFP-SCR reporter ES cells transiently co-transfected with I-SceI expression vector and with control vector (Control, orange or blue), F53BP1wt fragment ( F53BP1wt , maroon or dark blue), F53BP1D1521R fragment ( D1521R , apricot or grey), Luciferase control siRNA (si Luc , brown or teal) or SMARTpool siRNA against Exo1 (si Exo1 , light brown or sky blue). Paired t -test versus control in Brca1 Δ/mut cells —F53BP1wt : P =0.0001, D1521R : NS; in Brca1 fl/mut cells —F53BP1wt : NS, D1521R : NS. Paired t -test si Luc versus si Exo1 in Brca1 Δ/mut cells: P =0.00007, in Brca1 fl/mut cells: P =0.0001. Error bars indicate s.e.m. throughout. ( b ) Frequency of I-SceI-induced LTGC events in the same experiment as in panel ( a ). Paired t -test versus control in Brca1 Δ/mut cells —F53BP1wt : NS, D1521R : NS; in Brca1 fl/mut cells —F53BP1wt : NS, D1521R : NS. Paired t -test si Luc versus si Exo1 in Brca1 Δ/mut cells: P =0.001, in Brca1 fl/mut cells: P =0.007. ( c ) Ratio of I-SceI-induced GFP + RFP + /total GFP + frequencies (LTGC/overall GC, expressed as a percentage) from the same experiment as in panels ( a ) and ( b ). Paired t -test against control in Brca1 Δ/mut cells —F53BP1wt : P =0.0003, D1521R : NS; in Brca1 fl/mut cells —F53BP1wt : NS, D1521R : NS. Paired t -test si Luc versus si Exo1 in Brca1 Δ/mut cells: P =0.0001, in Brca1 fl/mut cells: P =0.007. ( d ) Abundance of 53BP1 fragments, Exo1 and actin (loading control) in treated Brca1 Δ/mut and Brca1 fl/mut RFP-SCR reporter ES cells in ( a ), ( b ) and ( c ). Full size image Brca1/CtIP controls the annealing step of SDSA The idea that a defect in DNA end resection could translate into a defect in late stages of HR seems paradoxical. We considered the hypothesis that the bias towards LTGC in Brca1 mutant cells is the consequence of failed termination of STGC. We tested this hypothesis by constructing a new ‘one-ended’ RFP-SCR reporter, in which the non-invading DNA end (marked with a red star in Fig. 6a ) lacks GFP sequences. I-SceI -induced STGC (GFP + RFP – ) occurring in this reporter cannot be terminated by homologous pairing (annealing), but must instead use non-homologous mechanisms to rejoin the displaced nascent strand with the non-invading, non-homologous second end of the DSB. 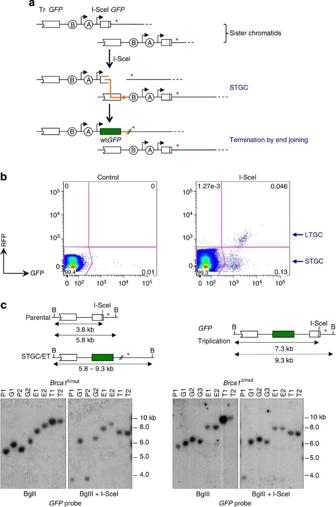Figure 6: Analysis of I-SceI-induced STGC and LTGC in ‘one-ended’ HR reporter cells. (a) Structure of the ‘one-ended’ RFP-SCR reporter. Circles A and B: 5′ and 3′ artificialRFPexons. TrGFP: 5′ truncatedGFP. Black arrows: promoters. Orange arrow: Rad51-mediated strand invasion (3′ end marked with arrow head). The second (non-invading) end of DSB lacksGFPsequences (marked with red star; compare withFig. 1a). The annealing step is not available to terminate STGC (GFP+RFP–) and STGC termination must occur by end joining. LTGC (GFP+RFP+) products are not shown. (b) Primary FACS data showing I-SceI-induced HR products inBrca1fl/mut‘one-ended’ RFP-SCR reporter ES cells. Note the I-SceI-induced GFP+RFP–(STGC) and GFP+RFP+(LTGC) populations. (c) Southern blot analysis of HR products in one-ended RFP-SCR reporter cells. ‘Parental’: unrearranged reporter; ‘ET’: ‘Early termination’ LTGC products. For ‘STGC/ET’ events, termination is predicted to occur by end-joining, producing HR products of varying size. ‘GFPtriplication’: LTGC product. B: Bgl II sites. I-SceI sites are marked, as are restriction fragment sizes. Red star: non-homologous second end of I-SceI-induced DSB. Boxes areGFPcopies; the green box is wtGFP.RFPcassette is not shown. gDNA from individual clones was digestedin vitrowith BglII alone or with BglII+I-SceI as shown; Southern blot membranes were probed withGFPprobe. The two left-hand panels (Brca1fl/mut) are taken from one gel. The two right-hand panels (Brca1Δ/mut) are taken from one gel. Gel lanes—P1–P2: parental clones; G1–G3: STGC (GFP+RFP–) clones; E1–E2: early termination LTGC (GFP+RFP+) clones; T1–T2: LTGC (GFP+RFP+) ‘GFPTriplication’ clones. Only ‘parental’ and ‘GFPtriplication’ clones contain an I-SceI site within the repaired reporter; this site is lost in the STGC and ET clones. The slight differences in gel mobility of the G1, G2, E1 and E2 bands between the two panels from theBrca1fl/mutgel reflect bowing of the gel during electrophoresis or Southern transfer. Figure 6: Analysis of I-SceI-induced STGC and LTGC in ‘one-ended’ HR reporter cells. ( a ) Structure of the ‘one-ended’ RFP-SCR reporter. Circles A and B: 5′ and 3′ artificial RFP exons. Tr GFP : 5′ truncated GFP . Black arrows: promoters. Orange arrow: Rad51-mediated strand invasion (3′ end marked with arrow head). The second (non-invading) end of DSB lacks GFP sequences (marked with red star; compare with Fig. 1a ). The annealing step is not available to terminate STGC (GFP + RFP – ) and STGC termination must occur by end joining. LTGC (GFP + RFP + ) products are not shown. ( b ) Primary FACS data showing I-SceI-induced HR products in Brca1 fl/mut ‘one-ended’ RFP-SCR reporter ES cells. Note the I-SceI-induced GFP + RFP – (STGC) and GFP + RFP + (LTGC) populations. ( c ) Southern blot analysis of HR products in one-ended RFP-SCR reporter cells. ‘Parental’: unrearranged reporter; ‘ET’: ‘Early termination’ LTGC products. For ‘STGC/ET’ events, termination is predicted to occur by end-joining, producing HR products of varying size. ‘ GFP triplication’: LTGC product. B: Bgl II sites. I-SceI sites are marked, as are restriction fragment sizes. Red star: non-homologous second end of I-SceI-induced DSB. Boxes are GFP copies; the green box is wt GFP . RFP cassette is not shown. gDNA from individual clones was digested in vitro with BglII alone or with BglII+I-SceI as shown; Southern blot membranes were probed with GFP probe. The two left-hand panels ( Brca1 fl/mut ) are taken from one gel. The two right-hand panels ( Brca1 Δ/mut ) are taken from one gel. Gel lanes—P1–P2: parental clones; G1–G3: STGC (GFP + RFP – ) clones; E1–E2: early termination LTGC (GFP + RFP + ) clones; T1–T2: LTGC (GFP + RFP + ) ‘ GFP Triplication’ clones. Only ‘parental’ and ‘ GFP triplication’ clones contain an I-SceI site within the repaired reporter; this site is lost in the STGC and ET clones. The slight differences in gel mobility of the G1, G2, E1 and E2 bands between the two panels from the Brca1 fl/mut gel reflect bowing of the gel during electrophoresis or Southern transfer. Full size image We targeted a single copy of the ‘one-ended’ RFP-SCR reporter to the ROSA26 locus of Brca1 fl/mut ES cells. We generated isogenic clones of Cre-treated Brca1 fl/mut one-ended RFP-SCR reporter cells that either had or had not undergone deletion of wt Brca1 . Consistent with the longer gene conversion (332 bp) required to produce GFP + products, we noted ~10-fold lower frequencies of I-SceI -induced STGC (GFP + RFP + ) products in Brca1 fl/mut cells compared to isogenic Brca1 fl/mut cells containing a conventional ‘two-ended’ RFP-SCR reporter ( Fig. 6b ); in contrast, the absolute frequencies of I-SceI-induced LTGC were little changed ( Fig. 6b ). Typically, about one-third of all measured HR products were GFP + RFP + , the remainder being GFP + RFP – ; this varied from clone to clone, the maximum LTGC:total HR ratio being ~60%. Southern analysis of FACS-sorted I-SceI-induced GFP + RFP – or GFP + RFP + populations derived from either Brca1 fl/mut or from Brca1 Δ/mut cells revealed STGC products of variable size, reflecting random termination by end joining ( Fig. 6c ); LTGC products revealed a combination of ‘early terminating’ LTGC (that is, LTGC with termination occurring between the two GFP copies of the donor) and ‘ GFP triplications’ ( Fig. 6c ). Consistent with the absence of an annealing step that can reliably terminate STGC, we noted a higher proportion of ‘early terminating’ LTGCs in one-ended reporter cells than in the original two-ended reporter cells: in Brca1 fl/mut one-ended RFP-SCR reporter cells, 6/21 (29%) of all LTGCs were early terminating and 15/21 (71%) were GFP triplications; in Brca1 Δ/mut one-ended RFP-SCR reporter cells, 9/23 (39%) of all LTGCs were early terminating and 14/23 (61%) were GFP triplications (difference between Brca1 fl/mut and Brca1 Δ/mut is not significant by χ 2 analysis). We noted reduced I-SceI-induced HR frequencies in four independent one-ended RFP-SCR reporter Brca1 Δ/mut clones, in comparison with four independent Brca1 fl/mut clones ( Fig. 7a ). However, HR in Brca1 Δ/mut one-ended RFP-SCR reporter cells revealed exactly proportionate reductions in STGC and LTGC, with no additional LTGC bias ( Fig. 7a ). Further, transient expression of wt BRCA1 in Brca1 Δ/mut one-ended RFP-SCR reporter cells restored both STGC and LTGC in equal proportions ( Fig. 7b ). Thus, in contrast to the conventional two-ended RFP-SCR reporter ( Fig. 3 ), in the context of the one-ended RFP-SCR reporter, STGC and LTGC are each equivalently Brca1 -dependent ( Fig. 7b ). Further, siRNA-mediated depletion of CtIP reduced STGC and LTGC in equal proportions in both Brca1 fl/mut and Brca1 Δ/mut one-ended RFP-SCR reporter cells and thus had no statistically significant impact on the STGC/LTGC balance ( Fig. 7c ). Therefore, when the annealing step of STGC is inactivated, loss of Brca1/CtIP has no impact on the relative balance between STGC and LTGC. 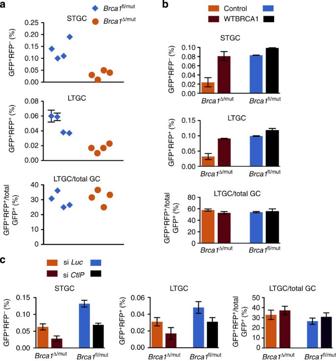Figure 7: BRCA1/CtIP fails to affect the STGC/LTGC balance if the annealing step of STGC termination is abolished. (a) I-SceI-induced HR in four independent Cre-treated one-ended RFP-SCR reporter ES cell clones of each genotype:Brca1fl/mut(blue diamonds) andBrca1Δ/mut(orange circles). Each point shows the mean of quadruplicate samples for one independent clone. Error bars: standard error of the mean (s.e.m.). If invisible, error bars are smaller than symbols. (b) Wild-type humanBRCA1complements both the STGC and LTGC defects inBrca1Δ/mutone-ended RFP-SCR reporter ES cells. Data pooled from three independent experiments, each performed in triplicate. Error bars: s.e.m.,n=3. Top panel: I-SceI-induced STGC inBrca1Δ/mutandBrca1fl/mutone-ended RFP-SCR reporter ES cells transiently transfected with I-SceI and with either control (orange or blue) or wtBRCA1(maroon or dark blue) expression vectors.Brca1Δ/mutcells: wtBRCA1versus control: pairedt-test:P=0.003.Brca1fl/mutcells: wtBRCA1versus control: NS. Middle panel: I-SceI-induced LTGC in the experiment shown in the top panel.Brca1Δ/mutcells: wtBRCA1versus control: pairedt-test:P=0.003.Brca1fl/mutcells: wtBRCA1versus control: NS. Bottom panel: Ratio of I-SceI-induced LTGC/overall GC in the experiment shown in the upper panels.Brca1Δ/mutcells: wtBRCA1versus control: NS.Brca1fl/mutcells: wtBRCA1versus control: NS. (c) CtIP depletion reduces STGC and LTGC in equal proportions in one-ended RFP-SCR reporter cells. Data pooled from three independent experiments, each performed with triplicate samples. Left panel: I-SceI-induced STGC inBrca1Δ/mutandBrca1fl/mutRFP-SCR reporter ES cells co-transfected with I-SceI and with either control Luciferase siRNA (siLuc, orange or blue bars) or CtIP SMARTpool (siCtIP, maroon or dark blue bars). Pairedt-test inBrca1Δ/mutcells:P=0.05; inBrca1fl/mutcells:P=0.02. Middle panel: I-SceI-induced LTGC in the same experiment. Pairedt-testBrca1Δ/mutcells:P=0.04; inBrca1fl/mutcells: NS. Right panel: Ratio of I-SceI-induced LTGC/overall GC in the same experiment. Pairedt-test inBrca1Δ/mutcells: NS; inBrca1fl/mutcells: NS. Figure 7: BRCA1/CtIP fails to affect the STGC/LTGC balance if the annealing step of STGC termination is abolished. ( a ) I-SceI-induced HR in four independent Cre-treated one-ended RFP-SCR reporter ES cell clones of each genotype: Brca1 fl/mut (blue diamonds) and Brca1 Δ/mut (orange circles). Each point shows the mean of quadruplicate samples for one independent clone. Error bars: standard error of the mean (s.e.m.). If invisible, error bars are smaller than symbols. ( b ) Wild-type human BRCA1 complements both the STGC and LTGC defects in Brca1 Δ/mut one-ended RFP-SCR reporter ES cells. Data pooled from three independent experiments, each performed in triplicate. Error bars: s.e.m., n =3. Top panel: I-SceI-induced STGC in Brca1 Δ/mut and Brca1 fl/mut one-ended RFP-SCR reporter ES cells transiently transfected with I-SceI and with either control (orange or blue) or wt BRCA1 (maroon or dark blue) expression vectors. Brca1 Δ/mut cells: wt BRCA1 versus control: paired t -test: P =0.003. Brca1 fl/mut cells: wt BRCA1 versus control: NS. Middle panel: I-SceI-induced LTGC in the experiment shown in the top panel. Brca1 Δ/mut cells: wt BRCA1 versus control: paired t -test: P =0.003. Brca1 fl/mut cells: wt BRCA1 versus control: NS. Bottom panel: Ratio of I-SceI-induced LTGC/overall GC in the experiment shown in the upper panels. Brca1 Δ/mut cells: wt BRCA1 versus control: NS. Brca1 fl/mut cells: wt BRCA1 versus control: NS. ( c ) CtIP depletion reduces STGC and LTGC in equal proportions in one-ended RFP-SCR reporter cells. Data pooled from three independent experiments, each performed with triplicate samples. Left panel: I-SceI-induced STGC in Brca1 Δ/mut and Brca1 fl/mut RFP-SCR reporter ES cells co-transfected with I-SceI and with either control Luciferase siRNA (si Luc , orange or blue bars) or CtIP SMARTpool (si CtIP , maroon or dark blue bars). Paired t -test in Brca1 Δ/mut cells: P =0.05; in Brca1 fl/mut cells: P =0.02. Middle panel: I-SceI-induced LTGC in the same experiment. Paired t -test Brca1 Δ/mut cells: P =0.04; in Brca1 fl/mut cells: NS. Right panel: Ratio of I-SceI-induced LTGC/overall GC in the same experiment. Paired t -test in Brca1 Δ/mut cells: NS; in Brca1 fl/mut cells: NS. Full size image This report documents a functional communication between BRCA1 and later stages of HR, as revealed by a bias towards LTGC when BRCA1 function is impaired. Expression of wild-type but not cancer-predisposing BRCA1 alleles restored the STGC/LTGC balance in Brca1 mutant cells, suggesting that BRCA1 performs a tumour suppressor function in this process. Depletion of the BRCA1-interacting end resection protein CtIP (or its activator, Sirt6) or of Exo1 mimicked or enhanced the Brca1 mutant STGC/LTGC imbalance. Further, inhibition of 53BP1, a key antagonist of the DNA end resection function of Brca1, normalized the STGC/LTGC balance in Brca1 Δ/mut cells. This suggests that defects in DNA end processing are the cause of the LTGC bias in Brca1 Δ/mut cells. To identify the mechanisms underlying this phenomenon, we studied STGC and LTGC within a new ‘one-ended’ reporter, in which STGC cannot be terminated by annealing. Surprisingly, in the context of the ‘one-ended’ reporter, although overall HR retained dependence on BRCA1 and CtIP, loss of BRCA1/CtIP no longer influenced the balance between STGC and LTGC. This suggests that BRCA1/CtIP influences the STGC/LTGC balance in the context of two-ended DSBs by facilitating the annealing step that normally terminates STGC—most likely, by ensuring efficient and timely processing of the second end of the DSB ( Fig. 8 ). 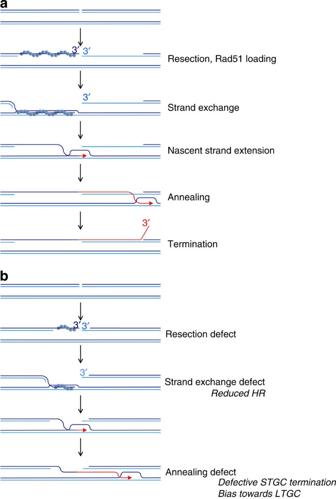Figure 8: Model: Brca1/CtIP acts on the second end of the DSB to promote the annealing step of SDSA. (a) SDSA in wild-type cells. Structural analysis of STGC inFigs 1cand6csuggests that the homologous second end of the DSB normally ‘edits’ short-tract gene conversions to a defined size. (b) In cells lacking Brca1/CtIP function, defective DNA end resection and impaired cooperation with Brca2/Rad51 results in a strand exchange defect. A defect in second-end resection leads to a relative impairment in the annealing step that normally terminates STGC. As a result, a higher proportion of HR events escape termination as STGCs and resolve as LTGCs. In the absence of a homologous second end of the DSB (such as in the ‘one-ended’ reporter—not shown in this figure), loss of Brca1/CtIP function has no impact on STGC termination and does not affect the STGC/LTGC balance. Figure 8: Model: Brca1/CtIP acts on the second end of the DSB to promote the annealing step of SDSA. ( a ) SDSA in wild-type cells. Structural analysis of STGC in Figs 1c and 6c suggests that the homologous second end of the DSB normally ‘edits’ short-tract gene conversions to a defined size. ( b ) In cells lacking Brca1/CtIP function, defective DNA end resection and impaired cooperation with Brca2/Rad51 results in a strand exchange defect. A defect in second-end resection leads to a relative impairment in the annealing step that normally terminates STGC. As a result, a higher proportion of HR events escape termination as STGCs and resolve as LTGCs. In the absence of a homologous second end of the DSB (such as in the ‘one-ended’ reporter—not shown in this figure), loss of Brca1/CtIP function has no impact on STGC termination and does not affect the STGC/LTGC balance. Full size image The SDSA model of somatic HR assumes an asymmetry between the two DNA ends, such that one end undergoes Rad51-mediated strand exchange and the second end does not ( Fig. 8 ) [7] . How asymmetry is established during SDSA is unknown; it could be imposed at several different stages, including the DNA end resection stage or during Rad51 filament assembly. Although the model proposed in Fig. 8 envisions a direct role for Brca1, CtIP and Exo1 in resection of the non-invading second end of the DSB, one or more of these proteins might also coordinate communication between the two DNA ends during end resection. Interestingly, recent work in Saccharomyces cerevisiae shows that the Mre11 nuclease and the CtIP homologue, Sae2, provide coordinated resection of the two ends of radiation-induced DSBs [50] . Currently, however, it is not possible to measure second-end resection or potential asymmetry between the two DNA ends in mammalian cells. Interestingly, the failure of Mre11 depletion to influence the STGC/LTGC balance suggests that not all mammalian complexes implicated in DNA end resection affect the balance between STGC and LTGC. In this regard, deletion of H2AX , an HR gene that can suppress DNA end resection in certain contexts [51] , does not appear to influence the STGC/LTGC balance [34] . Analyses of the impact of POL32 mutation on gap repair in S. cerevisiae [52] and in Drosophila melanogaster [53] suggest that SDSA may entail several different mechanisms of nascent strand extension that differ in their processivity and, hence, in their capacity to mediate LTGC. A major alternative model proposes that mammalian LTGC is mediated by a distinct copying mechanism, such as BIR. BIR may entail formation of a bona fide replication fork following strand exchange and therefore involves lagging strand synthesis [11] , [15] , [54] . A key trigger to BIR in yeast is a one-ended invasion occurring without a homologous second end [10] , [11] , [14] , [15] , [16] , [17] . In yeast, both RAD51 -independent and RAD51 -dependent forms of BIR are recognized [7] , [11] , [13] , [14] , [15] . RAD51 -independent BIR can act on short homologous sequences, tolerating homologies down to ~30 bp [55] . By analogy, a defect in DNA end resection and Rad51 loading in Brca1 mutants might lead to the formation of abnormal synapses that favour BIR—perhaps similar to the recently proposed idea of microhomology-mediated BIR (MM-BIR) [56] —leading to the observed LTGC bias in Brca1 mutants. We consider this BIR model of LTGC in detail below. In contrast to the avid engagement of BIR following chromosomal one-ended invasions in S. cerevisiae , the majority of chromosomal one-ended HR events in the mammalian system studied here resolve as STGCs, as revealed by the abundance of GFP + RFP – products in this setting. There is indeed a proportionate bias in favour of LTGC in the ‘one-ended’ reporter compared to the ‘two-ended’ reporter; however, the absolute frequencies of I-SceI -induced LTGC at the ROSA26 locus in Brca1 fl/mut cells are equal in the two reporters (~0.05%; compare the LTGC frequencies in Figs 2c and 7a ). Thus, a forced ‘one-ended’ invasion in mammalian cells does not preferentially trigger BIR. The major effect of a forced ‘one-ended’ invasion in our experiments is an ~10-fold reduction in the frequency of GFP + RFP – STGCs (compare STGC frequencies in Figs 2c and 7a ). Importantly, a gene conversion of at least 331 bp is required to generate GFP + recombinants within the ‘one-ended’ reporter. The Jasin and Nickoloff labs previously measured gene conversions (GCs) within a conventional ‘two-ended’ reporter in mammalian cells and observed that ~80% of all GCs are less than 58 bp in length [19] , [20] . This suggests that the majority of STGCs occuring within the ‘one-ended’ reporter studied here may have been terminated prior to conversion to wt GFP and are therefore not detectable as GFP + products. Our findings are consistent with DNA fibre analysis of mammalian cells recovering from replication arrest, in which Rad51-dependent HR repair of collapsed forks—presumably mediated by one-ended invasions—was not found to be associated with replication restart [57] . Importantly, a pure ‘replication fork’ BIR model of LTGC also fails to explain why LTGC should be relatively independent of BRCA1 in the ‘two-ended’ reporter ( Figs. 2 and 3 ), but fully BRCA1-dependent in the context of the ‘one-ended’ reporter ( Fig. 7a,b ). In contrast, an SDSA model of LTGC can readily account for this difference, as it invokes a defect of HR initiation in Brca1 mutant cells and, for the ‘two-ended’ reporter only, a defect of STGC termination by annealing ( Fig. 8 ). These two defects will have opposing effects on the absolute frequency of LTGC only in the context of the ‘two-ended’ reporter and might create the appearance that LTGC is BRCA1 -independent in this setting (as in Fig. 3 ). Notably, Rad51-mediated invasions can trigger BIR in Xenopus laevis egg extracts [58] and it seems likely that a proportion of LTGCs in mammalian cells are bona fide BIR products. However, definitive analysis must await the development of an assay in mammalian cells that reliably separates BIR-mediated LTGCs from SDSA-mediated LTGCs. A defect in annealing suggests a new mechanism underlying genomic instability associated with loss of BRCA1. In BRCA1 mutant cells, a higher proportion of HR events may escape the error-free annealing step of SDSA termination; these ‘functionally one-ended’ invasions will be obligatorily mutagenic. Thus, the BRCA1 -dependent annealing step of SDSA termination is likely an important bulwark against genomic instability and cancer. Interestingly, a recent sequencing analysis of breast cancer genomes revealed elevated frequencies of tandem gene segment duplications [59] . Conceivably, some of these rearrangements could be the result of inappropriate engagement of LTGC during DSB repair. Molecular biology and antibodies The RFP-SCR reporter was constructed by conventional cloning methods using modified ROSA26 targeting vectors [34] . Expression vector for h BRCA1 was pcDNA3β [60] . siRNA SMARTpools were purchased from Dharmacon. Antibodies used were: Brca1 (Santa Cruz and anti-human BRCA1 Ab MS110, 1:100), CtIP (Santa Cruz,1:50), Bard1 (Santa Cruz, 1:500), Mre11 (Novus, 1:6,000), Sirt6 (Abcam, 1:500), Exo1 (Santa Cruz, 1:500), β-actin (Abcam, 1:2,000) and influenza haemagglutinin epitope tag Ab (Santa Cruz, 1:1,000). Cells were lysed in RIPA buffer (50 mM Tris–HCl, pH 8.0, 250 mM NaCl, 0.1% sodium dodecyl sulphate, 1% NP-40 with protease and phosphatase inhibitors). Extracted protein was resolved by 4–12% bis–Tris SDS–PAGE (Invitrogen) and analysed by western blotting using the antibodies described above. Supplementary Figs S8–S15 show full gel images of western blots and of the one Southern blot shown in other figures. Cell lines and cell culture The Brca1fl/mut ES cell line (11CO/47T) was a kind gift from Dr Alan Ashworth [37] . ES cells were grown in ES medium on either MEF feeders or gelatinized plates. The RFP-SCR reporter was targeted by electroporating 2 × 10 7 Brca1 fl/mut ES cells with 20 μg of linearized targeting vector, followed by seeding in 60-cm plates with puroR feeders. Puromycin (0.5 μg ml −1 ) was added 24 h later and colonies were picked 5–7 days later. Brca1 fl/mut ES cells contain one mutant Brca1 allele encoding a truncated gene product and a second Brca1 allele (which is functionally wild type but harbours loxP sites flanking exons 22–24) that can be conditionally inactivated by Cre-mediated recombination. We generated multiple Brca1 -deficient ES clones by transient adenovirus-mediated Cre expression to delete the exons 22–24. Cell line U2OS was obtained from ATCC. Southern blotting gDNA was extracted from confluent ES cells on six-well plates (5–10 × 10 6 cells) using a Puregene DNA Isolation Kit (Gentra Systems). Southern blotting was performed with GFP cDNA or ROSA26 5′ probe. In all, 7.5–10 μg of gDNA was digested with the appropriate restriction enzyme and run overnight on 0.8% gel with 0.5 × TBE at 35 V. The DNA was transferred overnight onto nylon membrane in 1 M NaCl and 0.4 M NaOH. The membrane was prehybridized for 30 min and labeled with GFP cDNA or ROSA26 5′ probe overnight [34] . The membrane was then washed and developed by autoradiography. In all experiments, including U2OS cells containing a randomly integrated reporter, only clones containing one intact copy of the reporter were used. Supplementary Figs S8–S15 show full gel images of western blots and of the one Southern blot shown in other figures. Recombination assays 2 × 10 5 cells were transfected in suspension in 24-well plates with 0.5 μg pcDNA3β-myc NLS-I-SceI [22] or 0.5 μg control vector pcDNA3β using Lipofectamine 2000 (Invitrogen). GFP + and GFP + RFP + frequencies were measured 3 days post transfection by FACS using Becton Dickinson 5 Laser LSRII in triplicates and corrected for transfection efficiency and background events. (Transfection efficiency was measured simultaneously by parallel transfection with 0.05 μg wt GFP expression vector.) Typically ~2 × 10 5 total events were scored per sample. In the BRCA1 complementation experiments ( Fig. 3 ), rescue was optimal at low levels of exogenous BRCA1 expression vector (0.1 μg pcDNA3β- BRCA1 +0.4 μg pcDNA3β-myc NLS-I-SceI or control vector per well). For siRNA experiments, cells were transfected with 1 μl 20 μM (that is, 20 pmol) siRNA+0.3 μg of pcDNA3β-myc NLS-I-SceI (or control vector) per well. In Figs 3 , 4 , 5 , 6 , HR data represent the mean and standard error of the mean of three independent experiments. Statistical analysis was by two-tailed paired t -test (unknown variance). RT-qPCR analysis RNA was extracted using QIAGEN RNeasy Mini Kit (QIAGEN Sciences, MD). Analysis of first-strand cDNA was by Power SYBR Green RNA-toC T 1-Step Kit (Applied Biosystems, Foster City, CA). An ABI 7300 Real time PCR System was used for RT-qPCR. Taqman probe and primer sets to genotype for Brca1 were: Brca1 —Exon 22–23, sense: 5′-TTCCGTGGTGAAGGAGCTT-3′; Brca1 —Exon 22–23, antisense: 5′-TGGCTGCACGATCACAAC-3′; Brca1 —Exon 23–24, sense: 5′-GCCTGGACAGAAGACAGCA-3′; Brca1 —Exon 23–24, antisense: 5′-CAGTCCCACATCACAAGACG-3′. We used conventional SYBR green RT-qPCR assays of Gapdh and the siRNA-targeted gene. We used Primer 3 software (Whitehead Institute, MIT) to generate gene-specific primer sequences and confirmed use of each primer pair by melting curve analysis and gel electrophoresis. Primers used for RT–PCR: human BRCA1 —sense: TCACATGATGGGGAGTCTGA; human BRCA1 —antisense: TTCCCGATAGGTTTTCCCAAA; Brca1 —Exon 21–22, sense: ATGAGCTGGAGAGGATGCTG; Brca1 —Exon 21–22, antisense: CTGGGCAGTTGCTGTCTTCT; Brca1 —Exon 22–23, sense: GGTGCTCATCTAGTTGTGATCG; Brca1 —Exon 22–23, antisense: CTGTACCAGGTAGGCATCCA; Brca1 —Exon 7–8, sense: AGCCTAGGTGTCCAGCTGTC; Brca1 —Exon 7–8, antisense: CTGCAATCACCTGGCTTAGTT; CtIP —sense: ATGGTCAAGAATCTGAACCC; CtIP —antisense: TGAGGAGGTGTCTTTGAAGCAG; Bach1 —sense: ATCCGGTGTCAGAGATGTCC; Bach1 —antisense: CAAGGAGTAGAGCCCGTGAG; Rap80 —sense: GAAGGAAAACCCTCCTCCTG; Rap80 —antisense: TGTTCTTGGCCTCTCTTCGT. mRNA was measured in triplicates with a standard curve generated for each gene using cDNA obtained from each sample. The expression level of target genes was normalized to internal Gapdh . Cell cycle analysis ES cells were pulsed with 10 μM BrdU for 15 min, 48 h after transfection with siRNA, and fixed in 70% ethanol. BrdU was counterstained using anti-BrdU (Boehringer-Mannheim, 1:40) with a secondary FITC-conjugated rabbit anti-mouse antibody (Jackson Immuno Research, 1:50). After exposure to RNase and staining with propidium diiodide, approximately 10 4 events were acquired using a Becton Dickinson 5 Laser LSR II and the results were analysed using FloJo software. How to cite this article: Chandramouly, G. et al. BRCA1 and CtIP suppress long-tract gene conversion between sister chromatids. Nat. Commun. 4:2404 doi: 10.1038/ncomms3404 (2013).